The mechanism of ultrafast structural switching in superionic copper (I) sulphide nanocrystals Superionic materials are multi-component solids with simultaneous characteristics of both a solid and a liquid. Above a critical temperature associated with a structural phase transition, they exhibit liquid-like ionic conductivities and dynamic disorder within a rigid crystalline structure. Broad applications as electrochemical storage materials and resistive switching devices follow from this abrupt change in ionic mobility, but the microscopic pathways and speed limits associated with this switching process are largely unknown. Here we use ultrafast X-ray spectroscopy and scattering techniques to obtain an atomic-level, real-time view of the transition state in copper sulphide nanocrystals. We observe the transformation to occur on a twenty picosecond timescale and show that this is determined by the ionic hopping time. Superionic conductors are solids that exhibit a critical temperature above which their ionic conductivity is similar to those found in ionic liquids, with applications in electrochemical energy storage devices as solid-state electrolytes and as resistance switching devices [1] , [2] , [3] . Studied by Faraday [4] , superionic materials consist of a compound in which one species forms a rigid crystalline cage and another species occupies the interstices. Upon heating into the superionic phase, the rigid cage expands and often acquires new symmetry, permitting the second species to move freely within the fixed sublattice. Ionic conductivities approach 1 Ω −1 cm −1 , corresponding to ions moving between sites on the single picosecond timeframe [5] , [6] . Furthermore, many superionic materials exhibit a critical temperature close to ambient, increasing the technological applicability of this unique solid–liquid hybrid behaviour. For example, copper (I) sulphide exhibits superionicity above 103 °C, where the monoclinic sulphur lattice expands into a largely vacant hexagonal structure; the copper ions, for which there are many more sites than ions, abandon their fixed low-temperature positions and move freely among the many possible sites in the hexagonal sulphur lattice, displaying the characteristic high ionic conductivity of superionic phases [7] , [8] , [9] , [10] . Recent work in nanoscale superionics has shown that the transition temperature is reduced at small sizes and that polymer surface treatments enable stabilization of the superionic phase to room temperature [11] , [12] . Room-temperature superionic behaviour of lithium has recently been observed in Li 10 GeP 2 S 12 and can be stabilized close to room temperature in LiBH 4 , sparking increased interest in superionic materials for practical electrochemical devices [13] , [14] , [15] , [16] . Despite the long history of investigations into superionic materials, the mechanism of the structural reorganization and how that gives rise to high ionic conductivity remains largely unknown, especially at the nanoscale. As nanocrystals behave as single non-interacting domains, they are model systems for understanding phase transformations [17] . Molecular dynamics and other theoretical treatments have been applied to the study of the phase transition in a range of compounds, but have not considered nanoscale superionics [18] , [19] , [20] . Experiments on superionics for nanoscale resistance switching devices and non-volatile memory applications have observed switching on 100 μs time scales (refs 3 , 21 ). Recent transmission electron microscopy experiments have directly observed equilibrium fluctuations on few-second timescales between the low- and high-temperature phases in an individual Cu 2 S nanorod held at the critical temperature [22] . These studies report the time interval to stabilize a nucleus of the high-temperature phase close to the critical temperature but do not record the dynamic details of the structural transformation itself on the timescale on which the ions are moving. Here we present time-resolved X-ray spectroscopic and scattering studies probing the superionic phase transition in Cu 2 S nanodisks with femtosecond temporal resolution, permitting an atomic-level study of the superionic transformation capable of resolving the intrinsic atomic motion. These dynamic studies allow one to separate the emergence of superionic diffusional motion from the concomitant crystallographic change. We observe reversible switching between the low-temperature and high-temperature superionic phase in less than 20 ps, but significantly longer than the timescale of the temperature jump. These measurements are carried out in an excitation regime in which the thermal energy is comparable to the energy barrier between the two phases, such that the transformation time scale is determined by the intrinsic dynamics of the structural reorganization and not the probability of a nucleation event [20] , [23] . Picosecond near-edge X-ray spectroscopy Copper (I) sulphide nanodisks (10 nm diameter) were observed using ultrafast X-ray pump–probe techniques at beamline 6.0.2 at the Advanced Light Source (ALS) at Lawrence Berkeley National Laboratory [24] , [25] . Samples were photo-excited with above-band-gap 400 nm light pulses of 50 fs pulse duration. The incident fluence of 8 mJ cm −2 induced impulsive temperature jumps of approximately 570 °C above room temperature, which corresponds to a superheating of approximately 500 °C (the details of this calculation are presented in the Methods). The near-edge X-ray absorption fine structure (NEXAFS) spectrum at the copper L 3 absorption edge was then measured in transmission, allowing a study of the transient behaviour of the local copper bonding environment. Measurements of the copper L 3 NEXAFS spectrum probe the 2 p →3 d transition by promoting a core electron into an unoccupied state in the copper d band. As the copper core electrons contribute very little to inter-atomic bonding, changes in the L 3 spectrum are mainly due to changes in the copper d band. These measurements provide an ensemble-averaged probe of all copper sites within each nanocrystal and monitor the average copper bonding environment. 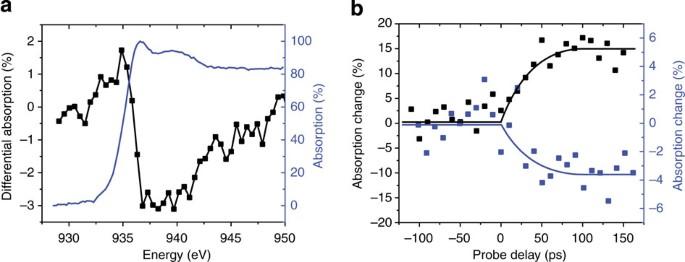Figure 1: Evidence of a spectral red-shift. (a) Observed differential energy spectrum at a probe delay of 400 ps (black) with the unexcited spectrum overlaid (blue). The differential spectrum corresponds to a red-shift of the spectrum. (b) Time traces at the two peak energies of the differential spectrum (935 eV in black, 937.5 eV in blue) confirm the spectral red-shift observed after time zero. The solid lines inbare guides to the eye. Figure 1a shows changes in the L 3 spectral shape at a time 400 ps after photo-excitation with the unexcited spectrum overlaid. The differential spectrum, generated by subtracting the laser-off spectrum from the laser-on spectrum, shows two pronounced features: a positive peak at 935 eV and a broader negative feature from 936 to 945 eV. The maximum of the low-energy peak in the differential energy trace occurs at the midpoint of the main L 3 edge, whereas the opposite-polarity trough is located above the main edge. Such features correspond to a subtle red-shift of the copper L 3 edge, with no other discernible changes to the spectral shape. Figure 1: Evidence of a spectral red-shift. ( a ) Observed differential energy spectrum at a probe delay of 400 ps (black) with the unexcited spectrum overlaid (blue). The differential spectrum corresponds to a red-shift of the spectrum. ( b ) Time traces at the two peak energies of the differential spectrum (935 eV in black, 937.5 eV in blue) confirm the spectral red-shift observed after time zero. The solid lines in b are guides to the eye. Full size image To ascertain the dynamics of the observed spectral evolution, the near-edge absorption as a function of time was recorded at strategic energies of 935 and 937.5 eV, which are the energies of the largest amplitude changes in the differential energy spectrum. Initial measurements were carried out using the standard X-ray time structure with 100 ps time resolution. As shown in Fig. 1b , the observed time traces corroborate the differential spectrum data. The polarity of the traces on and above the edge is opposite, which verifies a shift of the main edge to lower energy occurring on a time scale faster than 100 ps. Despite the rapid onset of the effect, the red-shift persists for hundreds of nanoseconds, as can be seen in Fig. 2a . Such behaviour is consistent with a light-induced structural transition and not electronic effects due to changes in occupation of the valence and conduction band states, which would be expected to decay on faster timescales associated with carrier recombination rates [26] . The many-nanosecond decay seen in the transient absorption is due to thermal diffusion of the laser-deposited energy, a slow process dependent on sample preparation parameters that limits the switching recovery time of the system. 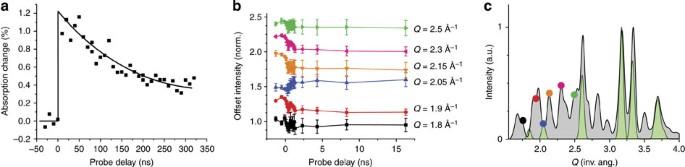Figure 2: Temporal evidence for a structural change. (a) Long-time recovery of the L3edge spectral red-shift showing several hundred nanosecond decay. The photon energy is 935 eV. (b) Time-resolved X-ray diffraction of Cu2S showing a photo-induced decrease in diffraction efficiency at severalQlocations, complemented by increased intensity of the high-temperature phase superionic (011) reflection (blue). Error bars signify the s.e. (c) Calculated powder diffraction patterns of nanocrystalline Cu2S in the high- and low-temperature phases. The reflections studied inbare marked with dots. Both low-temperature and high-temperature crystallographic standards (grey and green profiles, respectively) are corrected for isotropic nanocrystalline and instrumental broadening (from9). Figure 2: Temporal evidence for a structural change. ( a ) Long-time recovery of the L 3 edge spectral red-shift showing several hundred nanosecond decay. The photon energy is 935 eV. ( b ) Time-resolved X-ray diffraction of Cu 2 S showing a photo-induced decrease in diffraction efficiency at several Q locations, complemented by increased intensity of the high-temperature phase superionic (011) reflection (blue). Error bars signify the s.e. ( c ) Calculated powder diffraction patterns of nanocrystalline Cu 2 S in the high- and low-temperature phases. The reflections studied in b are marked with dots. Both low-temperature and high-temperature crystallographic standards (grey and green profiles, respectively) are corrected for isotropic nanocrystalline and instrumental broadening (from [9] ). Full size image Ultrafast X-ray diffraction To probe changes in the crystallographic symmetry, time-resolved X-ray diffraction measurements were performed at the Advanced Photon Source. The powder diffraction pattern was recorded as a function of probe delay under identical excitation conditions as the spectroscopic measurements. On account of the weak X-ray scattering of the nanocrystals, thick samples were studied, resulting in a smaller temperature elevation than in the absorption measurements. Consequently, although one cannot compare the onset behaviour of the diffraction effect to that of the X-ray absorption, these measurements provide further evidence that the observed changes in the absorption spectrum are associated with the superionic transformation. Owing to the finite-size broadening of the nanocrystalline sample, many of the finely spaced peaks, characteristic of the low-temperature phase, overlap to form broad features. Starting from the known crystallographic standards for the bulk low- and high-temperature phases, one may account for the finite-size broadening of a 10-nm crystallite and calculate theoretical nanocrystal diffraction patterns, resulting in Fig. 2c (refs 9 , 27 ). Supplementary Figure S1 shows the static sample diffraction pattern. One observes that many of the effective reflections from the monoclinic low-temperature phase vanish in the high-chalcocite phase, whereas the high-temperature phase has few reflections that do not strongly overlap with effective peaks of the broadened low-temperature pattern. As shown in Fig. 2b , the time-resolved measurements (black, red, orange, pink and green traces, also indicated in Fig. 2c ) show decreases in intensity by more than 15%, whereas a clear peak indexed to the high-temperature phase (blue trace) increases by a similar magnitude, indicating the expected change in crystallographic symmetry [12] , [22] . The full three-dimensional pattern may be seen in Supplementary Fig. S2 . The increase in intensity can be indexed to the (011) peak of the high-temperature hexagonal phase, consistent with previous work studying the thermally driven superionic phase transition in Cu 2 S (ref. 12 ). The large magnitude of the changes and the long-timescale recovery of the effect are consistent with the diffraction signature of the superionic phase transition in copper (I) sulphide. In addition, we note that the persistence of the time-resolved effect for many nanoseconds is in agreement with the long-lived spectral change seen at the copper L 3 edge. Femtosecond near-edge spectroscopy To overcome the limited time resolution of the time traces in Fig. 1 , femtosecond X-ray pulses were used to determine the rise time of the spectral red-shift at the energy of maximum amplitude. Femtosecond X-ray pulses were generated at the ALS using X-ray slicing techniques, in which a short X-ray pulse is sliced out of the long ~100 ps standard pulse, generating 200 fs full-width at half maximum pulses absolutely synchronized with the optical pump pulse. 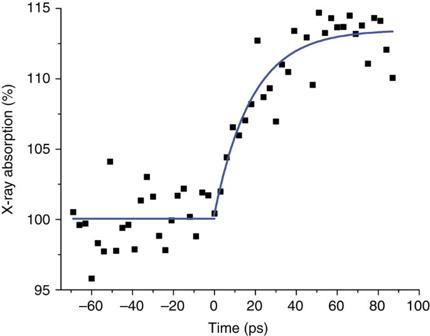Figure 3: Femtosecond resolution temporal evolution of L3edge shift. The time-resolved X-ray absorption at 935 eV is shown with 200 fs temporal resolution. The blue line is a single-exponential fit to the data with an 18 ps time constant. Figure 3 shows the measured dynamics at 935 eV, resolving the fundamental time scale for the red-shift in the NEXAFS spectrum. A single-exponential fit to the data reveals an ~18 ps onset time for the spectral evolution. This is significantly longer than the time scale for the temperature jump to occur, determined by electron–phonon coupling and carrier relaxation, which have been measured by optical pump–probe spectroscopy and shown in Supplementary Fig. S2 and [28] , [29] , [30] , [31] . It is also significantly longer than the time scale for acoustic propagation across the nanocrystal (a few picoseconds). This indicates a more complex transition mechanism than a simple thermal-expansion-driven process, which would be expected to occur on acoustically limited timescales [20] , [32] , [33] . Figure 3: Femtosecond resolution temporal evolution of L 3 edge shift. The time-resolved X-ray absorption at 935 eV is shown with 200 fs temporal resolution. The blue line is a single-exponential fit to the data with an 18 ps time constant. Full size image The high-temperature superionic crystal structure of copper (I) sulphide consists of a rigid, hexagonally close-packed lattice of sulphur atoms, with 2 copper atoms distributed randomly among 12 interstitial sites. Furthermore, the copper atoms have the ability to move between the interstitial sites and occupy the sites with equal probability, giving rise to superionicity. The low-temperature structure is a distortion of the superionic crystal, where the hexagonal symmetry of the sulphur lattice has been reduced to a monoclinic system as the volume of the unit cell contracts ( Fig. 4a ). The copper bonding then also distorts, and the ions assume a long-range order to their site occupancy in the monoclinic structure, eliminating high ionic conductivity. To understand how transforming from a the low-temperature monoclinic to the high-temperature hexagonal crystal structure would give rise to an L 3 red-shift, theoretical absorption spectra were generated using the ab-initio multiple-scattering X-ray absorption code FEFF [34] , [35] . FEFF-generated spectra of the high- and low-temperature phases were obtained directly from the atomic coordinates of all atoms within a given cluster, the atomic species, as well as an index marking unique atomic environments (see Methods). 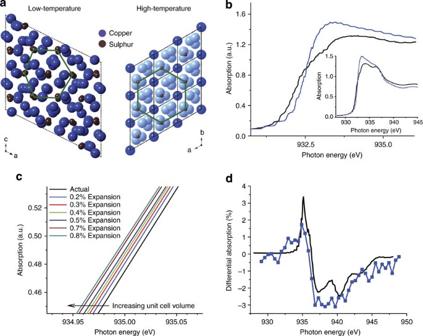Figure 4: Theoretical calculations of NEXAFS spectrum. (a) The theoretical treatment of NEXAFS spectra is based on the known crystal structures of the low-temperature and high-temperature crystal structures. The green hexagon marks the hexagonal-like symmetry maintained by the sulphur lattice in both phases. Note the overlapping copper sites of the high-temperature structure in light blue. (b) Simulated spectra of the two phases supports the conclusion that a red-shift occurs upon undergoing the superionic transformation. The high-temperature result is shown in black, with the low-temperature spectrum overlaid in blue. A broader view of the edge is shown in the inset. (c) The red-shift in L3edge position is found to be linear for small volume expansions (c), whereas the differential spectrum produced by approximating the transformation as a volume expansion of the low-temperature phase (black line) matches the experimental spectra (blue squares) quite well (d). Figure 4b shows calculated low- and high-temperature spectra at the copper L 3 edge using the known crystal structures as input. Although the dynamic partial-site occupancy of the high-temperature phase (represented as the light blue sites in Fig. 4a , which cannot be simultaneously occupied but are crystallographically equivalent) introduces complexities to the modelling, the transformation to the superionic configuration appears as a red-shift in the copper L 3 edge, further reinforcing the idea that the ultrafast spectral shift we observe is the signature of the superionic transformation. Figure 4: Theoretical calculations of NEXAFS spectrum. ( a ) The theoretical treatment of NEXAFS spectra is based on the known crystal structures of the low-temperature and high-temperature crystal structures. The green hexagon marks the hexagonal-like symmetry maintained by the sulphur lattice in both phases. Note the overlapping copper sites of the high-temperature structure in light blue. ( b ) Simulated spectra of the two phases supports the conclusion that a red-shift occurs upon undergoing the superionic transformation. The high-temperature result is shown in black, with the low-temperature spectrum overlaid in blue. A broader view of the edge is shown in the inset. ( c ) The red-shift in L 3 edge position is found to be linear for small volume expansions ( c ), whereas the differential spectrum produced by approximating the transformation as a volume expansion of the low-temperature phase (black line) matches the experimental spectra (blue squares) quite well ( d ). Full size image To develop a more intuitive understanding of how the known crystallographic changes of the phase transformation give rise to the spectral red-shift, NEXAFS spectra were calculated from the low-temperature crystal structure under various states of hydrostatic volume expansion. Note that the superionic phase transformation involves more crystal rearrangements than just volume expansion would impose. Also, the finite size of the nanocrystals introduces fine structure to the spectrum which the volume expansion approximation fails to capture. Still, such an approximation is motivated by the known volume increase of 0.7% associated with the superionic transition [8] . The low-temperature structure was used, because the atomic positions are well-defined and the superionic phase must evolve from the low-temperature structure in the experiment. Simulations were performed for a number of unit cell volume expansions, and the position of the main edge was found to red-shift linearly with the unit cell expansion for expansions less than 2% ( Fig. 4c ). A differential spectrum for comparison with the observed transient spectrum was generated by taking a 0.7% volume-expanded theoretical spectrum and subtracting the unexpanded theoretical spectrum, resulting in Fig. 4d . As these studies are intrinsically differential in nature, it is this calculated differential spectrum that is most valuable for comparison with experiment and captures the most salient features of the measured spectral changes, despite neglecting fine structure effects. The increased absorption at the main edge appears in the simulated difference spectrum with the same qualitative shape and width. The simulation also captures the decreased absorption just above the edge observed in the measured difference spectrum, as well as the recovery of the differential energy to zero in the vicinity of 947 eV. Also of note is that the approximate magnitudes of the calculated and observed effects are in order-of-magnitude agreement across the entire measured energy range. Although the thermal expansion dynamics at the experimental superheating may also contribute to expansion beyond that associated with the phase transformation, the good agreement of effect amplitude obtained using just the volume expansion associated with the phase transformation suggests that the structural rearrangement dominates the NEXAFS response. From this we conclude that the observed red-shift of the main edge corresponds to a lengthening of the copper bonds within the sample of a magnitude appropriate for the superionic transition. Although increased symmetry of the lattice upon transformation to the high-temperature phase does also alter the copper bond angles, which one might expect to alter the NEXAFS spectrum, it appears that the changed copper bond length contributes most strongly to the NEXAFS response. These results are in accordance with the well-established relationship between red-shifts in NEXAFS spectra and increases in bond length [36] . We now turn our attention to the time for the phase transition to occur. This is typically described by an Arrhenius/transition-state model, which is a function of an inverse attempt frequency and the probability of overcoming an activation barrier associated with the interface between the two phases [37] . We calculate the interfacial energy barrier to form a spherical nucleus of critical size (much smaller than a nanocrystal) to be about 100 meV, comparable to thermal energy fluctuations after laser excitation (70 meV), such that a large fraction of a nanocrystal has sufficient thermal energy to form the superionic phase. We therefore do not depend on thermal fluctuations to overcome the nucleation barrier. Although the system has a distribution of energies, we note that the thermal fluctuations at this superheating are such that even regions with thermal energy less than the activation barrier must only wait for approximately one attempt to surmount the barrier before success. The details of the energetic situation are given in the Methods section. Thus, in this superheated limit, the time scale for the superionic phase transition is not determined by the probability of nucleating, which is usually small for most experiments and dominates the temporal response. Rather, in this regime the nucleation probability approaches unity, and the transformation time is determined more strongly by the inverse attempt frequency, here associated with the time for the structure to rearrange, observed in this experiment to be about 20 ps. We note that this transformation time is comparable with the time for a copper ion to self-diffuse the length of a bond, in agreement with the known ionic diffusion coefficient of ~10 −6 cm 2 s −1 in the superionic phase [5] , [38] . The ionic self-diffusion process has a relatively small activation barrier, often attributed to a collective motion of the ionic system, which lowers the barrier for ionic hopping in the high-temperature phase [39] , [40] . The time for self-diffusion may itself be described with an Arrhenius model, where the coefficient of the exponential term represents the period of ionic motion in the material. For superionic conductors, the period of the coordinated cation motion has been determined by far-infrared and microwave studies to be ~1 ps (refs 6 , 39 ). Indeed, taking values for the energy barrier associated with the ionic hopping process in the superionic phase ( E a =240 meV), the inverse cation attempt frequency (1 ps), and treating the time to self-diffuse one hop in the simplest approximation as described by , one obtains a time comparable to that observed here experimentally [27] . As our experiment was performed on an ensemble of nanoparticles, the observed time represents the expected value of many events; this allows direct comparison between experiment and the calculated cation self-diffusion time. These measurements indicate that the time for the superionic transformation may be completely described by the average time for a successful copper ion self-diffusion event. That is to say that it is the ionic hopping time, which determines the fundamental time scale for the phase transition. As the superionic transformation requires no compositional change, and only a minor crystal rearrangement, such a conclusion is consistent with a transformation of the diffusionless class and a collective rearrangement of the nanocrystalline system. It is interesting to note that one may describe the superionic transformation dynamics using the material parameters of the high-temperature phase, indicating that the superionic transport properties emerge before the structure rearranges. In summary, by utilizing X-ray absorption and scattering techniques with femtosecond temporal resolution, we determine that the onset of superionicity in nanoscale copper (I) sulphide is governed by the time for the collective copper motion within a nanocrystal. These studies indicate a connection between the equilibrium transport properties in the superionic phase and the mechanism of the phase transformation itself, linking the short-range ionic displacements with the large-scale homogeneous crystallographic rearrangements of the nanocrystal, and providing a means of separating ionic and crystallographic degrees of freedom. More broadly, these studies demonstrate new means of using light to control the emergence of new phases and the speed at which these transformations occur. Future work may enable devices taking advantage of these ultrafast transformations for the development of resistive switching devices operating at the few-picosecond level. Preparation of nanocrystalline samples Stoichiometric copper (I) sulphide nanodisks, 10 nm in diameter and 2 nm thick, were prepared using a modified colloidal synthesis technique [41] . Samples were characterized using differential scanning calorimetry (DSC) to verify the reversibility of the transition and the critical temperature at the nanoscale. DSC was performed using a TA Instruments Q100 under nitrogen purge. The measurement was performed in accordance with the standard for determining phase-transition temperatures by DSC [42] . The measurement was repeated four times; the thermal cycle for the first three extended from 0 to 125 °C, whereas the fourth cycle continued up to 200 °C. The four thermal traces are shown in Supplementary Fig. S4a ; the traces overlap such that one cannot distinguish any cycle from any other cycle. From this data, we conclude that the superionic transition in superionic nanoparticles occurs at 77 °C with an approximate width of 5 °C. Furthermore, we note that the transformation is completely reversible and that the nanoparticles do not sinter at elevated temperature, which would be expected to shift the transformation temperature closer to the bulk value of 103 °C for subsequent thermal cycles [7] . The nanodisks were suspended in toluene and dropcast onto 100 nm thick silicon nitride membranes, which provide X-ray transparent sample support. Supplementary Fig. S4b shows a transmission electron micrograph of the copper (I) sulphide nanodisks. One can see both the top and side views. The disks tend to stand on end and stack, whereas the top view of the nanodisks may be seen on the right side of the image. To determine the rate of carrier relaxation after optical excitation, and hence the timescale of the resulting temperature increase, ultrafast optical and terahertz-frequency absorption measurements on the copper (I) sulphide nanodisks were performed. Samples were dropcast on optically transparent substrates to a sufficient thickness, so as to have an approximate optical density of one. The samples were then excited with ultrashort pulses of 400 nm light at a fluence of 8 mJ cm −2 , and the absorption of delayed THz and 800 nm pulses were recorded in transmission. The low photon energy of the THz photons does not allow for direct band gap excitation, but can be absorbed through intraband absorption by free electrons in the conduction band; this provides an extremely sensitive probe of free-carrier density. The 800-nm photons can also be absorbed by intraband excitation, providing a secondary free-carrier density probe, as well as a probe sensitive to changes in band structure. Ultrafast near-edge X-ray absorption X-ray absorption was measured by an avalanche photodiode placed in the transmitted X-ray beam with a 250-μm aluminium foil to prevent the detection of pump laser photons. The ALS is intrinsically pulsed with pulses every 2 ns of ~70 ps duration, and the avalanche photodiode was fast enough to resolve the few-nanosecond nature of the ring structure. The output was amplified using fast pre-amplifiers, such that the detection was sensitive to single X-ray photons, and gated so as to measure one X-ray pulse per excitation. A second reference X-ray pulse was measured ~1 ms after excitation, providing a laser-off reference. The gated signal was subsequently integrated on a shot-by-shot basis to generate laser-on and laser-off signals and improve acquisition quality. Each probe delay was recorded as the average signal over several seconds, and each time scan was repeated several times to achieve the necessary signal-to-noise ratio. The experiment has an absolute energy resolution of 0.9 eV. Measurements were also performed in a femtosecond X-ray mode, in which 200 fs full-width at half maximum X-rays were sliced from the standard X-ray bunch by a copropagating ultrashort laser pulse interacting with an electron bunch in an X-ray radiator, at the expense of a factor of ~10 4 in incident X-ray flux. These are subsequently dispersed spatially from the background picosecond X-rays, and slits are used to select the femtosecond X-rays, with a contrast ratio better than 2:1 at the Cu L 3 edge [43] , [44] . X-ray detection is the same as already described. The slicing laser pulse is absolutely synchronized in time to the sample excitation laser pulse. Time-resolved diffraction Samples were synthesized and excited identically to those used in the spectroscopic measurements. Samples were dropcast repeatedly to make a sample thick enough to scatter monochromatic 100 ps X-ray pulses of 8 keV energy (1.5 Å), resulting in a thicker sample than used for X-ray absorption measurements, which lessens the imposed temperature jump. The nanocrystal powder diffraction pattern was collected by a gated area detector in transmission. The incident X-ray spot size was less than 50 μm in diameter. Theoretical scattering patterns were calculated using the commercial Crystal Diffract software, accounting for a 10-nm diameter isotropic crystallite size and 0.003 Å −1 of instrumental broadening. The high-temperature phase calculation is based on International Centre for Diffraction Data (ICDD) reference 00–046–1195, which accounts for the dynamic partial site occupancy of that phase. FEFF near-edge spectrum simulations The absorbing atom in the cluster was explicitly specified. Different crystallographic sites were considered sufficiently unique environments to warrant unique indices. Models were run under the approximation of a fully screened core hole, which removes the dependence of unique potentials on the coordination shell relative to the absorbing atom. Clusters of ~275 atoms were used for both the low- and high-temperature phases, and established crystal structures were used to generate the atomic coordinates as shown in Fig. 3 and [7] , [8] , [9] , [45] . Previous work has shown that the high-temperature phase has copper sites too close to one another to be simultaneously occupied; consequently, a representative configuration was used that preserved the greatest number of different Cu–Cu and Cu–S bond lengths while adhering to this restriction. Furthermore, different absorbing sites were simulated, sampling various atomic sites, as well as the interior and surface of the atomic cluster. For each cluster/absorber combination, FEFF calculated an electronic band structure and the subsequent theoretical NEXAFS spectrum. The outputs for the different absorbers were then averaged to generate a spectrum comparable to experimental spectra. Energy calculations A calculation of the temperature of the nanocrystals after carrier thermalization, but before the onset of any phase transformation, provides the thermal-driving force for the phase transformation. Within the extinction depth of the light, the temperature increase caused in a material by an incident laser pulse may be described by the equation , where α (1.92 × 10 5 cm −1 ) is the optical cross-section, F is incident laser fluence (8 mJ cm −2 ), C is the specific heat (76.3 J/mol K) and N is the molar density [44] , [10] . Note that one does not include the latent heat of the superionic transformation when calculating the driving force temperature, as the low-temperature phase has only been superheated and has not yet transformed. To calculate the equilibrium temperature jump, one must include the latent heat, as well as the larger specific heat of the superionic phase (112 J/mol K) [10] . Inclusion of these effects indicates an equilibrium temperature jump of ~375 K, which is within the superionic phase stability region. Under the experimental conditions, the entire volume of a given nanocrystal is near-instantaneously (per the discussion of carrier thermalization presented in Supplementary Fig. S3 ) and homogeneously superheated, such that homogeneous nucleation may occur. Consequently, we consider only homogeneous nucleation. One may calculate the size of the high-temperature critical nucleus by considering the superheating calculated above and the expression , where T c is the superionic transition temperature, Δ H is the enthalpy of transformation, σ is the surface energy of the critical nucleus and Δ T is the superheating. We calculate σ by equating it to half of the enthalpy of melting a volume with that many bonds; that is to say that the dangling bonds on the embryo surface cost half of the energy of the bond in the bulk. This approximation is commonly made [46] , [47] . Consequently, we calculate a critical radius of 2.2 Å, yielding a critical energy of 90 meV per nucleus, comparable to kT . Note that we consider the activation barrier to be equal to the surface energy of the critical nucleus; we do not consider the volume energy decrease in the critical nucleus, as the atoms have not had sufficient time to rearrange, although their bonds have broken, creating a surface. Also note that the critical radius size is much smaller than the size of the nanocrystal itself. The fractional population of critical-nucleus-sized regions within one nanoparticle that have enough thermal energy to overcome this barrier may be expressed as after laser excitation, indicating these measurements are carried out in a superheated limit in which the energy required to form a critical nucleus is thermally available. Furthermore, if one were to consider the time for a cluster of atoms without sufficient energy to surmount the interfacial barrier due to thermal fluctuations, one calculates (ref. 22 ). Therefore, approximately one attempt to surmount the barrier is required to form a critical nucleus, even by the fraction of the nanocrystal that formally lacks the thermal energy to do so. How to cite this article: Miller, T.A. et al. The mechanism of ultrafast structural switching in superionic copper (I) sulphide nanocrystals. Nat. Commun. 4:1369 doi: 10.1038/ncomms2385 (2013).